Competing signals drive telencephalon diversity The telencephalon is the most complex brain region, controlling communication, emotion, movement and memory. Its adult derivatives develop from the dorsal pallium and ventral subpallium. Despite knowledge of genes required in these territories, we do not understand how evolution has shaped telencephalon diversity. Here, using rock- and sand-dwelling cichlid fishes from Lake Malawi, we demonstrate that differences in strength and timing of opposing Hedgehog and Wingless signals establish evolutionary divergence in dorsal–ventral telencephalon patterning. Rock dwellers exhibit early, extensive Hedgehog activity in the ventral forebrain resulting in expression of foxg1 before dorsal Wingless signals, and a larger subpallium. Sand dwellers show rapid deployment of Wingless, later foxg1 expression and a larger pallium. Manipulation of the Hedgehog and Wingless pathways in cichlid and zebrafish embryos is sufficient to mimic differences between rock- versus sand-dweller brains. Our data suggest that competing ventral Hedgehog and dorsal Wingless signals mediate evolutionary diversification of the telencephalon. Adult derivatives of the telencephalon are singularly important in evolution and neurological disease. The dorsal-most component (the cerebral cortex) is acutely enlarged in mammals [1] , and this expansion may have prefigured new forms of communication, reasoning and memory in human ancestors [2] . The ventral portion, collectively called basal ganglia, controls complex motion and emotion. All jawed vertebrates possess a telencephalon and share an embryological division into dorsal (the pallium) and ventral (subpallium) territories [3] . The parts of the telencephalon (that is, cortex and ganglia) integrate brain function via networks of excitatory and inhibitory neurons that originate from the pallium and subpallium, respectively [4] , [5] , [6] , [7] . Notably, a balance between pallium-derived excitatory neurons and inhibitory neurons from the subpallium is necessary for proper social and sensory function. In fact, misbalance between these neuronal types may be a common facet of heterogeneous syndromes like autism and schizophrenia [8] , [9] . Studies in model organisms elucidate how cellular and molecular processes construct the telencephalon and its dorsal/ventral (DV) derivatives [6] . The telencephalon develops under the influence of ventral Hedgehog (Hh) and dorsal Wingless (Wnt) signals [10] , [11] . These morphogens are part of distinct, interacting pathways that pattern the entire neural tube [12] . In the zebrafish, the transcription factor foxg1 mediates DV cross-talk between Hh and Wnt signals [13] . Specifically, shh induces the expression of foxg1 in the presumptive telencephalon at neurula stage. foxg1 is required for ventral telencephalic fate [14] , [15] and directly inhibits the dorsalizing effects of wnt8b in the dorsal midline [13] . Despite the importance of DV telencephalon specification in evolution and disease [7] , the mechanisms generating natural diversity in pallium and subpallium proportions are largely unknown. The evolutionary developmental pathways that shape regions of the telencephalon can be explored using cichlid fishes from Lake Malawi (East Africa). Despite large variation in brains and behaviours [16] , [17] , genomic differences among lineages, species and populations are small [18] , [19] . Malawi rock dwellers (locally and hereafter called ‘mbuna’) are strongly territorial and aggressive; they breed and feed at high density in complex three-dimensional habitats. Most mbuna eat algae from the substratum. Adult mbuna brains exhibit enlarged anterior components: telencephalon and olfactory bulbs [16] , [17] . Sand dwellers (locally called ‘utaka’, hereafter called non-mbuna) are less site-specific and less aggressive. They breed on seasonal leks where males build sand bowers to attract females. Many non-mbuna capture small prey using acute vision. Their brains are elaborated for more caudal structures: optic tecta, thalamus and eyes [16] , [17] . We show that partitioning of the telencephalon into pallial and subpallial domains differs in mbuna versus non-mbuna cichlids because of integrated divergence in Hh and Wnt signals, along DV and anterior–posterior (AP) developmental neuraxes. The differences that we observe between these two Malawi ecotypes are heterochronic and quantitative. Therefore, we experimentally antagonize and enhance Hh/Wnt signalling using small molecules, in multiple species of mbuna versus non-mbuna and the zebrafish, to mimic natural diversity. Our data demonstrate how variation in early development works to specify evolutionary diversification of forebrain structures. Telencephalon DV organization of mbuna and non-mbuna differs After the pallial–subpallial boundary (PSB) is established during stage 13 (late somitogenesis) [20] , and before telencephalon eversion (late pharyngula, stage 16), the pallium and subpallium can be visualized and measured in toto , in transverse section. Mbuna embryos possess proportionally larger subpallial, and non-mbuna exhibit the opposite, larger pallia (Student’s t -test, n =16 for each of mbuna and non-mbuna, t =17.218, P <0.001, Fig. 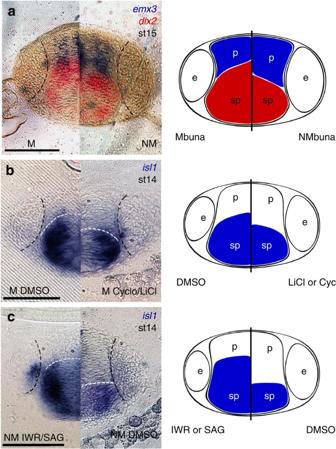Figure 1: Cichlid rock versus sand dwellers differ in pallial/subpallial proportions. (a–c) Left panels are transverse sections of the telencephalon at its greatest DV extent, and right panels are schematics of data depicted on the left. Black-dotted lines represent the position and size of the eyes in each section; note variance in eye size. Scale bar, 100 μm. (a) A ‘split-screen’ double ISH ofemx3(blue) anddlx2(red) used to visualize the pallium and subpallium in mbuna, left, and non-mbuna, right. (b) Expression of the subpallial markerisl1is depicted, and an expansion of the pallium (above dotted white line) in cyclopamine- or LiCl-treated mbuna (right side) versus DMSO control mbuna (left) is showed. (c) An expansion of the subpallium (below dotted white line) in SAG- or IWR-treated non-mbuna (left side) versus DMSO control non-mbuna (right) is showed. The treated specimens in summary panelsbandcare cyclopamine-treated mbuna and IWR-treated non-mbuna, respectively. 1a ; Table 1a shows data for three diverse species of mbuna and non-mbuna each, measured at stages 14 and 15). This can be nicely observed at stage 15 (equivalent to zebrafish prim-18), where the pallium is marked by emx3 expression and the subpallium by dlx2 . Figure 1a shows a transverse section through the telencephalon and uses a split-screen effect to demonstrate proportional differences between mbuna (left half-image) and non-mbuna (right half-image), assuming symmetry. Figure 1: Cichlid rock versus sand dwellers differ in pallial/subpallial proportions. ( a – c ) Left panels are transverse sections of the telencephalon at its greatest DV extent, and right panels are schematics of data depicted on the left. Black-dotted lines represent the position and size of the eyes in each section; note variance in eye size. Scale bar, 100 μm. ( a ) A ‘split-screen’ double ISH of emx3 (blue) and dlx2 (red) used to visualize the pallium and subpallium in mbuna, left, and non-mbuna, right. ( b ) Expression of the subpallial marker isl1 is depicted, and an expansion of the pallium (above dotted white line) in cyclopamine- or LiCl-treated mbuna (right side) versus DMSO control mbuna (left) is showed. ( c ) An expansion of the subpallium (below dotted white line) in SAG- or IWR-treated non-mbuna (left side) versus DMSO control non-mbuna (right) is showed. The treated specimens in summary panels b and c are cyclopamine-treated mbuna and IWR-treated non-mbuna, respectively. Full size image Table 1 Manipulation of Hh and Wnt signals changes cichlid and zebrafish pallial/subpallial compartments. Full size table Telencephalon divergence is mediated by Hh and Wnt signals We aimed to understand how evolutionary differences in the mbuna versus non-mbuna telencephalon are established. As cichlid embryos exit neurula stage, mbuna shh shows a larger DV domain, relative to non-mbuna, in its anterior-most area of expression ( Fig. 2a versus Fig. 2d ). By 4–5 somites, stronger shh activity in mbuna is correlated with foxg1 expression in the presumptive telencephalon ( Fig. 2e ). The non-mbuna shh domain is more ventrally restricted, expands dorsally more slowly and subsequent foxg1 in non-mbuna is delayed ( Fig. 2h ). Non-mbuna foxg1 is not expressed in the presumptive telencephalon until mid-stage 11 (8–10 somites). 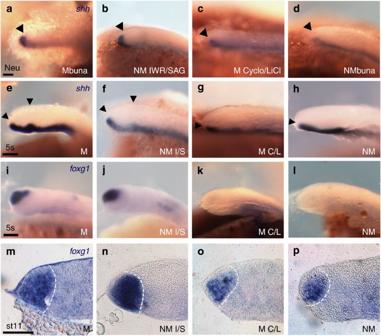Figure 2: Natural and experimental variation in the Hh and Wnt pathways modulates the pallial/subpallial gene circuit. (a–l) Images are lateral images of whole-mount embryos, anterior to the left. Neu ina–dand 5s ine–lrefer to neurula and five somite stages, respectively. Panelsm–pare midline, sagittal sections of embryos during late stage 11 (st11, 10–12 s). All panels from left to right are untreated mbuna (M), IWR- or SAG-treated non-mbuna (I/S), cyclopamine- or LiCl-treated mbuna (C/L) and untreated non-mbuna (NM). Specific treatments shown in the two summary (middle) columns are:b—IWR-treated (1 μM) NMbuna,c—cyclopamine-treated (50 μM) Mbuna,f—SAG-treated (1 μM) NM,g—LiCl-treated (1.25 M) M,j—SAG NM,k—cyclopamine M,n—IWR NM ando—LiCl M. Scale bar, 50 μm (applied to all four panels per row). (a–h) Arrowheads point to the dorsal progression ofshhexpression. (m–p) Dotted white lines outline the presumptive telencephalon. Figure 2: Natural and experimental variation in the Hh and Wnt pathways modulates the pallial/subpallial gene circuit. ( a – l ) Images are lateral images of whole-mount embryos, anterior to the left. Neu in a – d and 5s in e – l refer to neurula and five somite stages, respectively. Panels m – p are midline, sagittal sections of embryos during late stage 11 (st11, 10–12 s). All panels from left to right are untreated mbuna (M), IWR- or SAG-treated non-mbuna (I/S), cyclopamine- or LiCl-treated mbuna (C/L) and untreated non-mbuna (NM). Specific treatments shown in the two summary (middle) columns are: b —IWR-treated (1 μM) NMbuna, c —cyclopamine-treated (50 μM) Mbuna, f —SAG-treated (1 μM) NM, g —LiCl-treated (1.25 M) M, j —SAG NM, k —cyclopamine M, n —IWR NM and o —LiCl M. Scale bar, 50 μm (applied to all four panels per row). ( a – h ) Arrowheads point to the dorsal progression of shh expression. ( m – p ) Dotted white lines outline the presumptive telencephalon. Full size image Although mbuna elaborate Hh signalling along the DV axis, non-mbunas are characterized by increased Wnt activity along the AP axis. Like wnt1 , wnt8b progresses more rapidly from the midbrain–hindbrain boundary into the presumptive midbrain and diencephalon [17] . wnt8b enters the telencephalon at stage 11, following initial development of the pre-zona limitans intrathalamica [17] (pre-ZLI; Fig. 3 ). In non-mbuna, wnt8b is expressed in the telencephalon slightly before, or upon induction of foxg1 (7 somites); in mbuna, foxg1 has been expressed for approximately 10 h before wnt8b . Differences in the size of the foxg1 domain are apparent at this stage ( Fig. 2m ). The pallium and subpallium are then demarcated by the PSB at stage 13 ( Fig. 1 ). 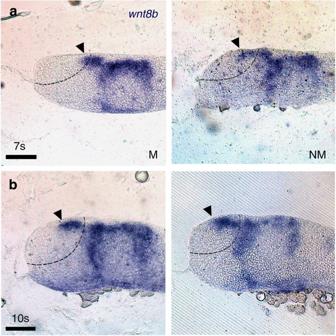Figure 3:wnt8bis first expressed in the cichlid telencephalon during mid-stage 11. For all panels, mbunas (Ms) are on the left, and non-mbunas (NMs) are on the right. Images are sagittal, midline sections. Scale bar, 50 μm. (a)wnt8bexpression is showed as it enters the telencephalon at 7 somites (7s). Arrows note the greater AP progression ofwnt8bexpression in NM versus M. (b)wnt8breaches its greatest AP extent in the telencephalon at 10s. Figure 3: wnt8b is first expressed in the cichlid telencephalon during mid-stage 11. For all panels, mbunas (Ms) are on the left, and non-mbunas (NMs) are on the right. Images are sagittal, midline sections. Scale bar, 50 μm. ( a ) wnt8b expression is showed as it enters the telencephalon at 7 somites (7s). Arrows note the greater AP progression of wnt8b expression in NM versus M. ( b ) wnt8b reaches its greatest AP extent in the telencephalon at 10s. Full size image Because of spatial and temporal differences in expression of Hh and Wnt ligands in cichlid telencephalon patterning [17] ( Fig. 2 ), we examined the activity of receptors and effectors in these pathways ( Fig. 4 ). As expected, in neurula and at 5 somites, ptc1 (a receptor for shh ) is expressed in the majority of the neural tube in mbuna, but is confined to a small ventral portion in non-mbuna ( Fig. 4b ). In model organisms, Gli3 integrates Hh and Wnt function. It is unclear what factors induce Gli3 in the forebrain [10] , but it is cleaved into a Hh-repressor form (Gli3R) where Hh activity is low [21] . Gli3R is a positive regulator of Wnt signalling in the forebrain [22] , [23] , and Wnt activates Gli3R specifically, via β-catenin [24] , [25] , [26] . Gli3R is necessary for proper specification of the pallium and this likely involves mutual repression of Hh [11] , and/or perhaps Foxg1 [13] . In cichlids, gli3 is pan-expressed in the anterior forebrain at neurula ( Fig. 4a ) but begins to recede dorsally in the presumptive telencephalon. In mbuna, foxg1 is induced, presumably by shh , at 4–5 somites ( Fig. 2 ) and is co-expressed with gli3 ( Fig. 4c ) for ~12 h (until stage 12, mid-somitogenesis). In non-mbuna, foxg1 is induced later ( Fig. 2 ) and gli3 expression takes longer to recede (the two are co-expressed until stage 13). Intriguingly, β-catenin, an effector of the canonical Wnt pathway, is upregulated 4–5 h before wnt8b expression in the telencephalon, and this upregulation occurs earlier in non-mbuna cichids ( Fig. 4e ). Note that β-catenin expression is grossly similar between mbuna and non-mbuna in more posterior serial sections from the same embryos ( Fig. 4e , grey arrow and inset images). 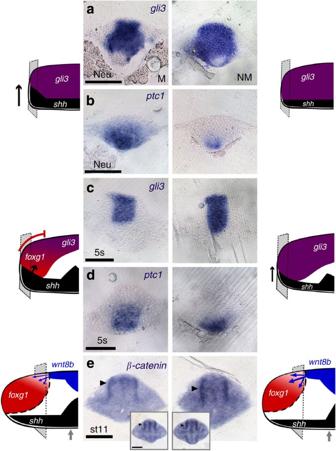Figure 4: Activity of the Hh and Wnt pathways during cichlid DV telencephalon patterning. Images are transverse sections of cichlid embryos. Scale bar, 50 μm. For all panels, mbunas (Ms) are on the left and non-mbunas (NMs) are on the right. At far left and right, schematics review the action of genes in the pallial/subpallial circuit (seeFig. 2) and show the position of the transverse sections (dotted grey rectangles). (a–d) Expression ofgli3, a mediator of Hh/Wnt signalling, andptc1, a receptor forshh, at neurula and 5 somites. (e) Activity of β-catenin in the forebrain during stage 11 (st11). Black arrowheads point to the DV signal of β-catenin in the dorsal telencephalon; the inset panels show β-catenin expression in the diencephalon; grey arrows in the schematics show the AP position of the inset panels. Figure 4: Activity of the Hh and Wnt pathways during cichlid DV telencephalon patterning. Images are transverse sections of cichlid embryos. Scale bar, 50 μm. For all panels, mbunas (Ms) are on the left and non-mbunas (NMs) are on the right. At far left and right, schematics review the action of genes in the pallial/subpallial circuit (see Fig. 2 ) and show the position of the transverse sections (dotted grey rectangles). ( a – d ) Expression of gli3 , a mediator of Hh/Wnt signalling, and ptc1 , a receptor for shh , at neurula and 5 somites. ( e ) Activity of β-catenin in the forebrain during stage 11 (st11). Black arrowheads point to the DV signal of β-catenin in the dorsal telencephalon; the inset panels show β-catenin expression in the diencephalon; grey arrows in the schematics show the AP position of the inset panels. Full size image Manipulation of Hh and Wnt signals mimics mbuna versus non-mbuna Our comparative data suggest that mbuna versus non-mbuna pallial/subpallial proportions differ due to quantitative changes in Hh and Wnt signalling. To test this hypothesis, we used small-molecule activators and antagonists to manipulate the Hh and Wnt pathways in both mbuna and non-mbuna embryos. Treatment of mbuna embryos with 50 μM cyclopamine, a Hh antagonist, for a brief window during neurula, knocks down shh expression and slows its progression dorsally during somitogenesis ( Fig. 2c ); this treatment phenocopies shh expression in non-mbuna. Conversely, treatment of non-mbuna embryos with the Hh agonist smoothened agonist (SAG) (1 μM) during neurula causes an expansion of shh expression in early somitogenesis, mimicking mbuna embryos ( Fig. 2b ). Notably, treatment of mbuna embryos with the Wnt activator lithium chloride (LiCl) (1.25 mM) phenocopies both the cyclopamine mbuna morphants and non-mbuna embryos, whereas treatment of non-mbuna with the Wnt antagonist inhibitor of Wnt response 1 (IWR-1) (1 μM) phenocopies the SAG non-mbuna morphants and mbuna embryos ( Fig. 2b ). Upregulation of Hh (SAG treatment) and downregulation of Wnt (IWR treatment) are sufficient to induce foxg1 earlier in non-mbuna morphants, whereas downregulation of Hh (cyclopamine) and upregulation of Wnt (LiCl) in mbuna morphants reproduce the delayed expression of foxg1 observed in non-mbuna embryos ( Fig. 2j ). Treatments at neurula stage similarly phenocopy differences in size of the foxg1 expression domain between mbuna and non-mbuna at stage 11 ( Fig. 2n ). Finally, we investigated the effect of treatment (again at neurula) on pallial/subpallial proportions 48 h later, during stages 14 and 15. Manipulation of either Hh (cyclopamine-treated, n =17, versus dimethylsulphoxide (DMSO) controls, n =13, t =14.468, P <0.001; SAG, n =11, versus DMSO, n =8, t =9.574, P <0.001) or Wnt (LiCl, n =14, versus DMSO, n =13, t =14.540, P <0.001; IWR, n =9, versus DMSO, n =8, t =8.629, P <0.001) pathways is sufficient to change pallial/subpallial organization from mbuna to non-mbuna proportions, and vice versa ( Fig. 1b ; Table 1a shows percentages for multiple neurula-treated mbuna and non-mbuna species). By varying the timing of manipulation with small molecules, we illustrate a narrow window of sensitivity for cross-talk between ventral and dorsal signals. Treatment of mbuna with cyclopamine after neurula (for example, during early somitogenesis) does not alter the onset of foxg1 expression, nor does it result in a larger pallium. Similar temporal specificity applies to non-mbuna; SAG treatment during somitogenesis does not induce earlier foxg1 expression, nor does it expand the subpallium. Conversely, upregulation of Wnt (LiCl) in mbuna phenocopies non-mbuna as long as treatment occurs before the induction of foxg1 at 4–5 somites. However, the effect of Wnt antagonism (IWR) in non-mbuna diminishes if treatment occurs after neurula stage. This time line implicates a factor that (i) limits the efficacy of Hh manipulation after neurula stage, (ii) responds flexibly to Wnt signals, (iii) but can act independently of them. We suggest that mbuna and SAG/IWR-treated non-mbuna possess a telencephalon that has been ventralized by Hh signal acting through early foxg1 expression to counteract dorsalizing factors. In contrast, non-mbuna and cyclopamine/LiCl-treated mbuna possess a telencephalon that has been dorsalized by gli3/Wnt activity that precedes foxg1 expression. To explore the generality of our treatment results, we manipulated pallial/subpallial proportions in the zebrafish. We first quantified pallial and subpallial volumes in wild-type (WT) zebrafish prim-18 stage (equivalent to stage 15 cichlids). The pallial percentage for zebrafish is comparable to values observed in non-mbuna ( Table 1b ). As in cichlids, an increase in Wnt signal (Student’s t -test, 0.2 M LiCl, n =5, versus DMSO controls, n =6, t =4.819, P <0.001; 4 μM 6-bromoindirubin-3′-oxime, n =7, versus DMSO, n =6, t =4.367, P <0.001) or a decrease in Hh activity (pooled 12 and 24 μM cyclopamine-treated, n =11, versus DMSO, n =6, t =3.860, P <0.001) is sufficient to expand the pallium at the expense of subpallium ( Table 1b ). In addition, zebrafish embryos were injected with shh mRNA at the 1–2 cell stage to increase Hh. Measurements at prim-18 show an expansion of the subpallium, similar to proportions observed in mbuna and SAG-treated non-mbuna cichlids (pooled 20, 40 and 80 pg of injected shh zebrafish morphants, n =17, versus WT controls, n =10, t =10.824, P <0.001, Table 1b ; Fig. 5 ). Finally, downregulation of the Wnt pathway via a dominant-negative tcf3 HS-activated construct [13] similarly results in a telencephalon with expanded subpallium (dnTcf3HS morphants, n =8, versus HS controls, n =7, t =4.68, P <0.001, Table 1b ; Fig. 5 ). Taken together, our manipulative experiments suggest that ventral Hh and dorsal Wnt signals interact to pattern the pallium and subpallium across bony fishes, despite differences in the timing of pathway activity between cichlids and zebrafish. 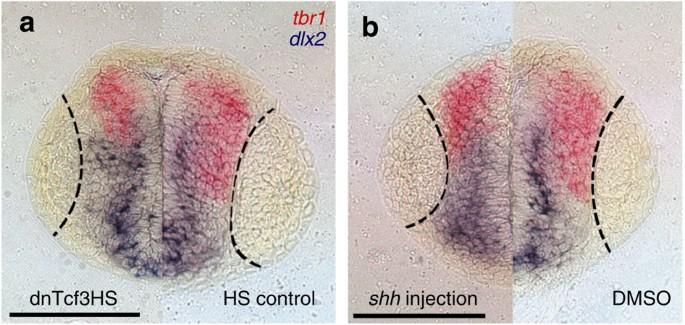Figure 5: Manipulation of Hh and Wnt signalling affects pallial/subpallial proportions in the zebrafish. Panels are frontal sections ofD. rerioembryos, showing the telencephalon at its greatest DV extent. Embryos are collected 32 h post fertilization or prim-18. Black-dotted lines represent the position and size of the eyes in each section; note variance in eye size. Scale bar, 100 μm. Bothaandbare split-screen double ISH oftbr1(red) anddlx2(blue), used to visualize the pallium and subpallium, respectively. (a) The effect of HS-activated dominant-negativetcf3(dnTcf3HS) is showed, an effector of the Wnt pathway (left side), compared with HS controls (right). (b) Split screen of an embryo injected at the one- to two-cell stage with 20 pgshhmRNA (left side) compared with a WT control (WT, right). These treatments (↓Wnt, ↑Hh) mimic mbuna cichlids (seeFig. 1). Figure 5: Manipulation of Hh and Wnt signalling affects pallial/subpallial proportions in the zebrafish. Panels are frontal sections of D. rerio embryos, showing the telencephalon at its greatest DV extent. Embryos are collected 32 h post fertilization or prim-18. Black-dotted lines represent the position and size of the eyes in each section; note variance in eye size. Scale bar, 100 μm. Both a and b are split-screen double ISH of tbr1 (red) and dlx2 (blue), used to visualize the pallium and subpallium, respectively. ( a ) The effect of HS-activated dominant-negative tcf3 (dnTcf3HS) is showed, an effector of the Wnt pathway (left side), compared with HS controls (right). ( b ) Split screen of an embryo injected at the one- to two-cell stage with 20 pg shh mRNA (left side) compared with a WT control (WT, right). These treatments (↓Wnt, ↑Hh) mimic mbuna cichlids (see Fig. 1 ). Full size image Cichlid and zebrafish brains develop at different rates, and this comparison is informative for models of telencephalon patterning. For instance, in the zebrafish, shh reaches the ventral presumptive telencephalon (anterior medial neural plate) first, immediately followed by foxg1 ; wnt8b appears in the telencephalic roof by 5–6 somites [13] . Cichlids show a greater time lag in the appearance of these molecules and dual heterochronic variation between mbuna and non-mbuna, along both DV and AP neuraxes ( Fig. 6a ). A simple model to explain telencephalon divergence between mbuna and non-mbuna begins with the initial difference in shh expression at neurula and the concomitant heterochrony in foxg1 expression ( Fig. 6a ). Note that the cichlid wnt8b promoter possesses vertebrate-conserved binding sites for foxg1 (ref. 13 ). The lag in timing between cichlid shh and foxg1 expression suggests that Hh signals may not induce foxg1 directly, and/or that a threshold of Hh/Gli complex activity is required for induction [13] . 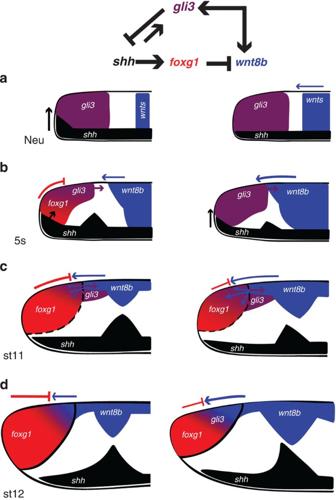Figure 6: Competing Hh and Wnt signals drive divergent pallial/subpallial patterning. At top, we illustrate the gene network that establishes pallial/subpallial proportions (see also Ulloa and Marti12). Arrows indicate positive signal; T bars indicate negative interactions. For all panels, mbunas are on the left, and non-mbunas are on the right. All schematics are lateral, midline representations. Neu, neurula; 5s, 5 somites; st11, stage 11 (6–12 somites); st12, stage 12 (13–20 somites). (a) Greater DV progression ofshhexpression in mbuna versus greater AP deployment of Wnt in non-mbuna. (b) Increasedshhin mbuna leads to earlier induction offoxg1, by 4–5s.gli3is present in the presumptive telencephalon of mbuna and non-mbuna, counteracted byfoxg1in mbuna only. (c) Aswnt8benters the telencephalon, mbunafoxg1has been established for some time. Non-mbunafoxg1is first expressed in the telencephalon slightly afterwnt8b. (d) Early elaboration offoxg1in mbuna andgli3/wnt8bin non-mbuna establishes contrasting readouts of ventralizing versus dorsalizing signals, at stage 12. Figure 6: Competing Hh and Wnt signals drive divergent pallial/subpallial patterning. At top, we illustrate the gene network that establishes pallial/subpallial proportions (see also Ulloa and Marti [12] ). Arrows indicate positive signal; T bars indicate negative interactions. For all panels, mbunas are on the left, and non-mbunas are on the right. All schematics are lateral, midline representations. Neu, neurula; 5s, 5 somites; st11, stage 11 (6–12 somites); st12, stage 12 (13–20 somites). ( a ) Greater DV progression of shh expression in mbuna versus greater AP deployment of Wnt in non-mbuna. ( b ) Increased shh in mbuna leads to earlier induction of foxg1 , by 4–5s. gli3 is present in the presumptive telencephalon of mbuna and non-mbuna, counteracted by foxg1 in mbuna only. ( c ) As wnt8b enters the telencephalon, mbuna foxg1 has been established for some time. Non-mbuna foxg1 is first expressed in the telencephalon slightly after wnt8b . ( d ) Early elaboration of foxg1 in mbuna and gli3 / wnt8b in non-mbuna establishes contrasting readouts of ventralizing versus dorsalizing signals, at stage 12. Full size image Because Wnt ligands do not enter the cichlid telencephalon until stage 11, our observations from comparative expression and small-molecule treatments (at neurula) require an early acting, anti-Hh factor, sensitive to induction by Wnt/β-catenin. We suggest that gli3 serves this role and that, in particular, Gli3R acts first (before 7–8 somites) as an early dorsalizing factor and then later as a dorsal analogue of ventral foxg1 , integrating Hh and Wnt signals to pattern telencephalic diversity ( Fig. 6 ). Overall, Hh and Wnt morphogens compete for influence along the DV axis of the entire brain, throughout ontogeny [11] , [12] , [27] . For example, it has been shown that eye loss and elaboration of the ventral forebrain in cavefish is partly explained by expansion of midline shh expression [28] , [29] . We demonstrate here how natural variation in telencephalon patterning evolves via temporal, spatial and quantitative tuning of both the Hh and Wnt pathways along integrated DV and AP neuraxes. Notably, our data combined with an earlier report [17] , suggest that, at least in Malawi cichlids, a large subpallium is the by-product of a large telencephalon, precisely because the evolutionary differences that we identify commence early in development. In the six mbuna and non-mbuna species that we studied, each have unique adult brains [16] , [17] , but exhibit little heterogeneity within groups at patterning stages. This implies an early neural blueprint for rock versus sand dwellers that is later elaborated for species-specific lifestyles and ecologies. Embryonic differences in the size of telencephalic compartments may thus facilitate, and also constrain variation in neuronal specification, sensory performance and social biology [30] , [31] . Telencephalon measurements Volumes of pallial and subpallial compartments were measured by integrating over transverse sections of the telencephalon in staged embryos of mbuna and non-mbuna species. Mbuna species included Cynotilapia afra (planktivore), Labeotropheus fuelleborni (algivore) and Maylandia zebra (generalist); non-mbuna species included Aulonocara jacobfreibergi (‘sonar’ hunter), Copadichromis borleyi (planktivore) and Mchenga conophoros (insectivore/generalist). We measured embryos at stages 14 and 15, following the first point (stage 13) [17] , [20] at which the pallium and subpallium can be distinguished by cellular boundaries (for example, the PSB). Proportions are consistent across stages 13–15, until telencephalon eversion (stage 16). We used gene expression to help visualize the PSB and telencephalic compartments: the pallium can be marked by pax6 , emx3 or tbr1 expression, and the subpallium by dlx2 or isl1 (see below for in situ hybridization (ISH)). Measurements were made using ImageJ on scaled images of transverse sections. We used morphological landmarks (for example, the anterior commissure ventrally and the epithalamus dorsally) to maintain consistency across individuals and species. Between 10 and 20 individuals (from multiple broods), per species were sectioned and prepared for measurement. To simplify analysis, individuals with oblique sections were eliminated, leaving 4–6 individuals per species. Pallial and subpallial measurements were expressed as a percentage of the total telencephalon. As the telencephalon encompasses more than one sequential transverse section, we used the Cavalieri method [32] (Σ (area of each section) * (distance between sections)) to express volumetric percentages. In situ hybridization ISH experiments are based on previously published protocols for cichlids [33] . Probes were constructed from cDNA sequences derived from partial genome assemblies of Lake Malawi cichlids [19] . The RNA probes are identical across the cichlid species used in this study. All ISH experiments were performed with multiple specimens (multiple individuals within single broods, then repeated at least twice with alternative broods) to fully characterize expression patterns within and across species. Once ISH was complete, embryos were embedded in gelatin-albumin blocks and sectioned [17] . Manipulation with small molecules Embryos from three mbuna species L. fuelleborni , M. zebra and C. afra were treated with LiCl, an activator of the Wnt pathway, or cyclopamine, an antagonist of the Hh pathway. The LiCl 1 M stock solution and 1.25 mM working concentration were prepared as described in Sylvester et al . [17] A 5 mM cyclopamine stock was used to obtain the final working concentration of 50 μM. Complementary experiments were performed using non-mbuna species A. jacobfreibergi , C. borleyi and M. conophoros . Embryos were treated with a Hh agonist, SAG (Enzo Life Sciences) [34] , or a Wnt antagonist, IWR-1 (Enzo Life Sciences) [35] . Stock and working concentrations for both SAG and IWR are 100 and 1 μM, respectively. Embryos in broods (one brood consists of 20–40 individuals) from each species of mbuna and non-mbuna were treated during neurula stage (approximately 36–40 h post fertilization) for 5 h at 28 °C, and bathed with either a chemical or DMSO vehicle controls (0.125% for LiCl; 1% for cyclopamine, SAG and IWR). Experiments were repeated with 2–4 additional broods for each species. After treatment, embryos were washed twice with fish water, placed in culture flasks with fresh fish water and incubated at 28 °C until they reached the desired stage. Treatment and control embryos were post-processed (ISH, sectioning and measurements) identically to descriptions above for untreated embryos. Additional experiments were conducted into early somitogenesis to identify the temporal window of sensitivity to treatment. Danio rerio experiments and processing WT zebrafish embryos were cultured in embryo media E2, then treated from bud to five somite stage with 1% DMSO and one of the following chemicals: 0.2 M LiCl (BDH Chemicals) or 4 μM 6-bromoindirubin-3′-oxime (Sigma-Aldrich) to promote Wnt/β-catenin signalling; or 12/24 μM cyclopamine (Sigma-Aldrich) to inactivate Hh. Embryos were washed twice with E2 and then incubated until prim-18 (32 h.p.f. at 28.5 °C). They were then fixed in 4% paraformaldehyde for 4 h at room temperature or overnight at 4 °C and afterwards washed with PBS and stored in methanol at −20 °C. In addition to treatment with small molecules, gene levels were manipulated directly. To downregulate Wnt signal, transgenic (Hsp70:ΔTcf3-GFP) [13] embryos were heat shocked at the tailbud stage for 30 min at 37 °C, incubated at 28 °C and fixed at prim-18. To upregulate Hh signal, shh mRNA for microinjection was prepared by digesting pSP64T-shh with Bam HI and transcribing with Sp6 polymerase (Ambion). The RNA was subsequently purified using the RNeasy kit (Qiagen), and 20, 40 or 80 pg was injected into one- to two-cell stage embryos. Embryos were cultured until prim-18 and fixed in paraformaldehyde as above. Embryos were then stained for dlx2 and tbr1 expression via double ISH to visualize and measure pallial–subpallial proportions as described for cichlid embryos (see above). How to cite this article: Sylvester, J. B. et al . Competing signals drive telencephalon diversity. Nat. Commun. 4:1745 doi: 10.1038/ncomms2753 (2013).